Patterned prevascularised tissue constructs by assembly of polyelectrolyte hydrogel fibres The in vivo efficacy of engineered tissue constructs depends largely on their integration with the host vasculature. Prevascularisation has been noted to facilitate integration of the constructs via anastomosis of preformed microvascular networks. Here we report a technique to fabricate aligned, spatially defined prevascularised tissue constructs with endothelial vessels by assembling individually tailored cell-laden polyelectrolyte hydrogel fibres. Stable, aligned endothelial vessels form in vitro within these constructs in 24 h, and these vessels anastomose with the host circulation in a mouse subcutaneous model. We create vascularised adipose and hepatic tissues by co-patterning the respective cell types with the preformed endothelial vessels. Our study indicates that the formation of aligned endothelial vessels in a hydrogel is an efficient prevascularisation approach in the engineering of tissue constructs. Cell survival within implanted engineered constructs depends on the timely formation of distributed, anastomosed vasculature [1] , [2] , [3] . Timely integration of the constructs with the host vasculature is important for providing oxygen and essential nutrients and for the removal of metabolic waste products [2] . Viable cells also require blood circulation within close proximity as the diffusion limit is ~100–200 μm [2] , [3] , [4] . There is thus a need to create prevascularised tissue-engineered constructs that facilitate rapid and directed anastomosis. The creation of a preformed microvascular network within a tissue construct has been successful in promoting vascular integration with the host [1] , [4] , [5] . These networks have been shown to rapidly anastomose with host vasculature, overcoming the problems posed by the slow ingrowth of physiological vasculature. Prevascularisation is generally achieved by seeding or encapsulating endothelial cells (ECs) with other cell types. However, in many of these approaches, the distribution of vasculature within a thick construct relies on in vitro cellular infiltration and self-organization of the cell mixture. These cellular processes are slow and the resultant vascularisation of the tissue construct is not uniform. Furthermore, the need for a critical concentration of ECs for the vascular self-assembly to occur in vitro severely limits the number of other cells that can be co-cultured [6] . One approach is to co-pattern ECs with other cell types in a hydrogel. The patterning of ECs in a prevascularised construct would serve to guide the distribution of the newly formed vasculature while simultaneously allowing the localization of ECs in defined regions at the critical density, leaving in the rest of the tissue construct space available for other cell types. Moreover, placing cells within hydrogels instead of creating completely cell-dense tissue constructs would provide an initial reservoir of nutrients to the encapsulated cells while allowing further diffusion of the required nutrients. However, co-patterning multiple cell types within a hydrogel is not a simple task. Cells have been patterned in three-dimensional (3D) hydrogels using techniques such as dielectrophoretic force cell patterning [7] , laser-guided direct writing [8] , micromolding of cell-laden hydrogels [9] and organ printing [10] . However, these techniques are limited by slow cell aggregation, the need for large volumes of cell suspension, complicated multistep processes and expensive instrumentation [11] . As a result, large-scale production of implantable 3D cell-patterned constructs at high resolution remains a challenge. Furthermore, these approaches have, to date, not successfully addressed the problem of vascularisation and mass transport through thick engineered tissue constructs [12] . Thus, our goal is to develop a scalable technique to build 3D cell-patterned constructs for creating vascularised tissues. An attractive encapsulation technique to create cell-laden hydrogel fibres is interfacial polyelectrolyte complexation (IPC) [13] , [14] . The advantage of this encapsulation technique is that the fibres are produced under aqueous conditions at room temperature [13] . The fibres are therefore amenable to the incorporation of biologics, including cells and proteins [14] . Subsequently, each cell-laden fibre can be used as a building block to create complex tissue constructs. In the present study, we develop an IPC fibre assembly technique to create an aligned endothelial vessel network that anastomoses with the host vasculature in a mouse model. Cell-laden fibres can also be assembled into highly patterned multicellular constructs. Patterned constructs of ECs with adipocytes and hepatocytes anastomose with the host, leading to vascularised tissues. This technique provides an easily adaptable platform to create 3D cell-patterned hierarchical structures that are spatially well defined and supported by vasculature, leading ultimately to functionally enhanced tissues. Assembly of cell-laden polyelectrolyte fibres Individual fibres were drawn in parallel from polyionic droplets arranged on a template and then assembled into higher-order structures ( Fig. 1a ). Fusion of these fibres was attained via secondary complexation, resulting in a continuous yet heterogeneous matrix ( Supplementary Fig. S1 ) that could be easily handled ( Supplementary Movie 1 ). The importance of being able to create individual niches at high resolution in a 3D environment has been recognized [15] , [16] , and we have achieved this by incorporating biologics in the polyionic solutions prior to drawing them into the fibres ( Fig. 1b,c ). Viability of encapsulated cells using this technique is generally high, with cells able to migrate and proliferate within the fibres (see Supplementary Fig. S2 and Supplementary Movies 2 and 3 ). 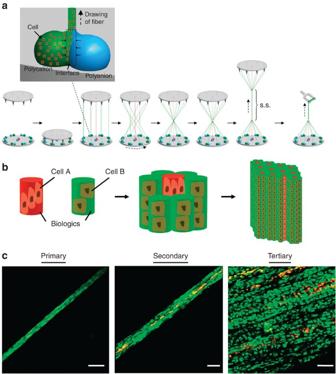Figure 1: Engineering of hierarchical tissue structures by fibre assembly. (a) Schematic of the process flow to achieve the hierarchical tissue structure at each step. Polyionic solutions containing biologics are first localized on a template. IPC fibres are drawn in parallel and brought to fuse at a single point by rotation of the template. Continuous upward drawing coupled with fusion by a deposited droplet of polyionic solution (either polycation or polyanion) forms the secondary structure (s.s.). The secondary structure is subsequently assembled to tertiary structure by spooling and layering secondary polyelectrolyte complexation. (b) Micropatterned niche environment can be created by assembling primary biostructural units containing different cell types. Each secondary structure consists of one central fibre surrounded by other fibres. This micropattern is repeated in the eventual tertiary construct. (c) Confocal microscopy images of the biostructural units. Labelled cells are encapsulated at high density in chitin–alginate polyelectrolyte fibres, demonstrating primary, secondary and tertiary structures. Scale bars: 100 μm. Figure 1: Engineering of hierarchical tissue structures by fibre assembly. ( a ) Schematic of the process flow to achieve the hierarchical tissue structure at each step. Polyionic solutions containing biologics are first localized on a template. IPC fibres are drawn in parallel and brought to fuse at a single point by rotation of the template. Continuous upward drawing coupled with fusion by a deposited droplet of polyionic solution (either polycation or polyanion) forms the secondary structure (s.s.). The secondary structure is subsequently assembled to tertiary structure by spooling and layering secondary polyelectrolyte complexation. ( b ) Micropatterned niche environment can be created by assembling primary biostructural units containing different cell types. Each secondary structure consists of one central fibre surrounded by other fibres. This micropattern is repeated in the eventual tertiary construct. ( c ) Confocal microscopy images of the biostructural units. Labelled cells are encapsulated at high density in chitin–alginate polyelectrolyte fibres, demonstrating primary, secondary and tertiary structures. Scale bars: 100 μm. Full size image Alignment of cells in fibre constructs To create an organized network of endothelial vessels within the hydrogel, we first investigated the processes of cell alignment and self-assembly to form tubes within the fibres. To demonstrate the use of fibres to align cells, we assembled IPC fibre constructs from the complexation of water-soluble chitin (WSC) and rat methylated collagen (RMC) with sodium alginate to form a continuous hydrogel with fibrous features and a uniform distribution of RMC ( Supplementary Fig. S3a,b ). We showed the alignment of ECs along the fibre axis. Similar observations were made with several other cell types. ( Supplementary Fig. S3b–e and Supplementary Movie 3 ). We have also studied neural stem cell (NSC) alignment and differentiation in our constructs. Fibre constructs with encapsulated NSCs were cultured in neural differentiation medium. After 10 days, we observed parallel alignment of NSCs. Additionally, positive staining for neurofilaments indicated in situ differentiation of NSCs within the construct ( Supplementary Fig. S3f ). In a further study, we observed tube morphogenesis of encapsulated Madin–Darby canine kidney cells when cocultured with NIH3T3 fibroblasts ( Supplementary Fig. S4a ). This behaviour was not observed in a control Madin–Darby canine kidney monoculture system ( Supplementary Fig. S4b ). The formation of parallel tube tracts indicated that the aligned collagen component within the matrix had directed the tube formation along the fibre axis. Formation of endothelial vessel network in IPC hydrogel We hypothesized that by assembly of EC-laden IPC fibres, we would be able to achieve patterning of an aligned vascular network within a gel matrix. We proceeded to investigate fibre constructs made up of repeating units that contained a central human EC-laden fibre for the ability to develop and maintain an endothelial vessel network in vitro and in vivo ( Fig. 2a ). Human mesenchymal stem cells (hMSCs) were used as mural cells to stabilize the endothelial vessels [17] , [18] . The formation of aligned endothelial tubes was observed within 24 h when cultured in vitro , which was verified at Day 7 by immunofluorescence staining for human von Willebrand factor (hVWF)-positive endothelial structures within our construct flanked by basement membrane protein—collagen type IV (Col IV) ( Fig. 2a and Supplementary Movies 4 and 5 ). These endothelial tubes, when co-encapsulated with hMSCs, remained stable for up to 56 days ( Supplementary Fig. S5 ). 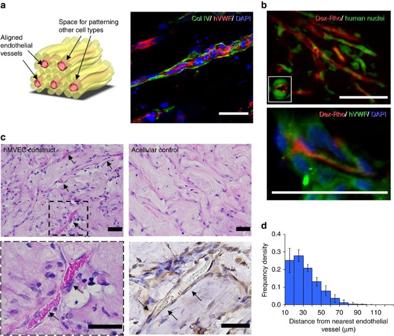Figure 2: Endothelial vessel network formation in fibre construct. (a) Schematic diagram illustrating the concept of a prevascularized hydrogel. Adjacent fibres could be used to pattern other cell types around the vessels.In vitroconfocal microscopy showed hVWF-positive (red) hMVECs aligned vessels with basement membrane collagen Type IV (Col IV) (green) in the fibre construct on Day 7. (b) Tail vein-injected dextran rhodamine was observed within the explanted hMVEC/hMSC constructs on Day 14, indicating that the endothelial vessels anastomosed with host vasculature. These vessels were surrounded by cells that stained positive for human nuclei and hVWF. (c) H&E-stained images of explanted hMVEC-laden construct on Day 28 (top left). Area within the dotted box is magnified (bottom left). Perfused vessels containing red blood cells (arrows) could be observed within the hMVEC-laden constructs on Day 28, but these vessels were notably absent in the acellular control (top right). Positive peroxidase staining for human CD31 (hCD31) shows that the implanted hMVEC formed a part of the endothelial vessels (arrows) within the fibre construct (bottom right). (d) Quantitative analysis of the hCD31-stained images shows that every location in the fibre construct section is <100 μm away from the nearest endothelial vessels (n=3). Scale bar: 50 μm. Figure 2: Endothelial vessel network formation in fibre construct. ( a ) Schematic diagram illustrating the concept of a prevascularized hydrogel. Adjacent fibres could be used to pattern other cell types around the vessels. In vitro confocal microscopy showed hVWF-positive (red) hMVECs aligned vessels with basement membrane collagen Type IV (Col IV) (green) in the fibre construct on Day 7. ( b ) Tail vein-injected dextran rhodamine was observed within the explanted hMVEC/hMSC constructs on Day 14, indicating that the endothelial vessels anastomosed with host vasculature. These vessels were surrounded by cells that stained positive for human nuclei and hVWF. ( c ) H&E-stained images of explanted hMVEC-laden construct on Day 28 (top left). Area within the dotted box is magnified (bottom left). Perfused vessels containing red blood cells (arrows) could be observed within the hMVEC-laden constructs on Day 28, but these vessels were notably absent in the acellular control (top right). Positive peroxidase staining for human CD31 (hCD31) shows that the implanted hMVEC formed a part of the endothelial vessels (arrows) within the fibre construct (bottom right). ( d ) Quantitative analysis of the hCD31-stained images shows that every location in the fibre construct section is <100 μm away from the nearest endothelial vessels ( n =3). Scale bar: 50 μm. Full size image Next, we implanted these endothelial constructs subcutaneously into mice with severe combined immunodeficiency (SCID) after 24 h of in vitro culture. To demonstrate that the endothelial vessels anastomosed with the host vasculature, dextran rhodamine dye was injected into the tail vein of the mouse on Day 14. Aligned vessels containing dextran rhodamine dye were observed in the explanted tissue construct ( Fig. 2b ). The presence of human nuclei- and hVWF-positive cells around these vessels indicated that the engineered vessels in the fibre-assembled hydrogel had integrated with the host vasculature ( Fig. 2b ). Histological analysis of constructs explanted on Day 28 showed that the acellular control construct exhibited minimum cell infiltration and an absence of vessel-like structures ( Fig. 2c ). In contrast, the endothelial construct demonstrated preservation of endothelial vessel structures with the infiltration of red blood cells (RBCs) ( Fig. 2c ). Uniform distribution of these RBCs containing endothelial vessels was observed within the implanted constructs ( Supplementary Fig. S6 ). The presence of the implanted ECs lining the vessels in our explanted EC-laden constructs was confirmed by human-specific CD31 staining ( Fig. 2c ). Moreover, patterning cells around the aligned endothelial tubes in a secondary structure guaranteed the close proximity of each cell to a vascular element below the 200-μm threshold distance associated with mass transfer limitations ( Fig. 2d and Supplementary Fig. S7 ). Hence, patterning EC within a hydrogel led to the formation of a prevascularised bed with patterned, perfused blood vessels. Engineering prevascularised adipose tissues We evaluated the ability of the fibre constructs to support the differentiation of 3T3-L1 adipocyte precursor cells over the course of 18 days, and the maintenance of EC-derived vascular structures during this time frame. We observed the formation of lipid vesicles in the differentiated 3T3-L1 cells encapsulated within the fibres ( Fig. 3a,b ). When co-patterned with ECs, adiponectin-positive cells aggregated around hVWF-positive endothelial tubes ( Fig. 3c,d ). We also embedded these coculture constructs within permissive RGD-QGel matrices and observed the sprouting of tubular structures into the gel, indicating the permissiveness of the fibre construct for eventual construct integration and anastomosis ( Supplementary Fig. S8 ). For implantation, 3T3-L1 cells were encapsulated within EC-laden constructs. The coculture constructs were differentiated for 18 days, after which they were implanted subcutaneously into SCID mice. Anastomosis of the engineered vascularised adipose tissue construct was indicated by the presence of aligned endothelial vessels with RBCs ( Fig. 3e ). The implanted adipocytes have the characteristic honey-comb appearance under hematoxylin and eosin (H&E) staining, with the presence of lipids confirmed via oil red O staining ( Fig. 3f ). 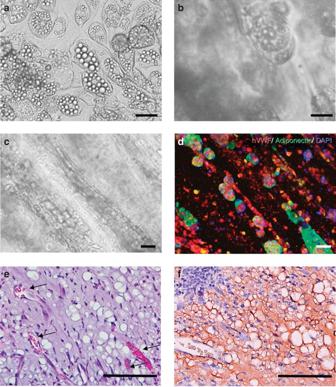Figure 3: Engineering of prevascularised adipose tissue. The accumulation of lipid vesicles after 18 days in both (a) tissue culture plate control and (b) within the fibres was used as an indicator for differentiation. (c) Tubulogenesis of EC in the constructs was evaluated using a central fibre laden with EC and 3T3-L1 in a 5:1 ratio surrounded by blank fibres. Tubulogenesis was observed after 2 days. (d) Immunostaining of human hVWF (red) with adiponectin (green) and DAPI (blue) confirmed the preservation of the endothelial vessels with closely associated clusters of differentiated 3T3-L1 after 18 days in culture. (e) Endothelial vessel formation within 3T3-L1/ EC coculture. H&E staining shows aligned patent blood vessels in close association with adipocytes within the fibre matrix, with arrows indicating the blood vessels. (f) Oil red O staining confirmed the presence of lipids. Scale bars: 100 μm. Figure 3: Engineering of prevascularised adipose tissue. The accumulation of lipid vesicles after 18 days in both ( a ) tissue culture plate control and ( b ) within the fibres was used as an indicator for differentiation. ( c ) Tubulogenesis of EC in the constructs was evaluated using a central fibre laden with EC and 3T3-L1 in a 5:1 ratio surrounded by blank fibres. Tubulogenesis was observed after 2 days. ( d ) Immunostaining of human hVWF (red) with adiponectin (green) and DAPI (blue) confirmed the preservation of the endothelial vessels with closely associated clusters of differentiated 3T3-L1 after 18 days in culture. ( e ) Endothelial vessel formation within 3T3-L1/ EC coculture. H&E staining shows aligned patent blood vessels in close association with adipocytes within the fibre matrix, with arrows indicating the blood vessels. ( f ) Oil red O staining confirmed the presence of lipids. Scale bars: 100 μm. Full size image Engineering prevascularised hepatic tissues Hepatic tissue is another tissue type that requires vascularisation [8] . To demonstrate the use of the endothelial vessel network to support liver function in vitro , we patterned primary rat hepatocytes and ECs at a high cell density in a secondary structure similar to the native liver sinusoid ( Fig. 4a ) and compared cellular morphology and functional maintenance to a control hepatocyte monoculture system. A niche microenvironment was created for the hepatocytes by incorporating galactosylated WSC in the hepatocyte fibres. Galactose is known to enhance hepatocyte function via a receptor-mediated mechanism [19] , [20] , [21] . The hepatocytes in the monoculture system were uniformly distributed throughout the fibre construct ( Fig. 4b ). In contrast, the hepatocytes in the coculture system aggregated around the ECs ( Fig. 4b ), agreeing with a previous report indicating the hepatocyte recruitment by endothelial vascular structures [11] . Albumin and CYP3A4 assays demonstrated improved maintenance of differentiated hepatocyte function when cocultured with ECs in a galactosylated niche ( Fig. 4c ). In controls without galactose, the in vitro function of the hepatocytes was not maintained ( Supplementary Fig. S9 ). These results suggested that the presence of the endothelial vessel network supported hepatocyte culture in vitro . 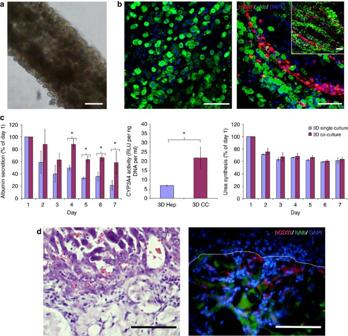Figure 4: Engineering of prevascularised hepatic tissue. (a) Bright-field microscopic image of a hepatocyte-laden fibre construct showing high cell density. (b) Immunostaining of hepatocyte monoculture (left) and coculture (right) with HUVEC after 24 h in fibre construct. Regions of aligned sinusoid-like structures were observed for the coculture. Hepatocytes and HUVEC were stained positive with rat serum albumin (rAlb) and hVWF, respectively. (c) Functional characterization of hepatocyte cultures. Better maintenance of albumin secretion function and higher CYP3A4 activity were observed for the co-culture construct. Urea synthesis function for both constructs remained relatively stable over 7 days. * denotes intergroup significant difference (P<0.01) at the specific time point (n=3, mean±s.d.). (d) H&E-stained and immunostained images of explanted hESC-derived hepatocyte constructs. Immunostaining indicates the presence of human serum albumin (hAlb)-positive cells in close association with hCD31-positive endothelial cells. Tissue scaffold boundary is indicated by white dotted line. Scale bars: 100 μm. Figure 4: Engineering of prevascularised hepatic tissue. ( a ) Bright-field microscopic image of a hepatocyte-laden fibre construct showing high cell density. ( b ) Immunostaining of hepatocyte monoculture (left) and coculture (right) with HUVEC after 24 h in fibre construct. Regions of aligned sinusoid-like structures were observed for the coculture. Hepatocytes and HUVEC were stained positive with rat serum albumin (rAlb) and hVWF, respectively. ( c ) Functional characterization of hepatocyte cultures. Better maintenance of albumin secretion function and higher CYP3A4 activity were observed for the co-culture construct. Urea synthesis function for both constructs remained relatively stable over 7 days. * denotes intergroup significant difference ( P <0.01) at the specific time point ( n =3, mean±s.d.). ( d ) H&E-stained and immunostained images of explanted hESC-derived hepatocyte constructs. Immunostaining indicates the presence of human serum albumin (hAlb)-positive cells in close association with hCD31-positive endothelial cells. Tissue scaffold boundary is indicated by white dotted line. Scale bars: 100 μm. Full size image We also patterned human embryonic stem cells (hESCs)-derived hepatocyte precursor cells (HPCs) with ECs to create vascularised hepatic tissues. After 5 days in culture, the coculture constructs were implanted into SCID mice in the liver after partial hepatectomy for 14 days. We observed the presence of the hESC-derived HPCs by immunostaining against human albumin, with vascularisation indicated by the hCD31 stain ( Fig. 4d ). Our approach of assembling fibres in a spatially defined manner, which allows for patterning of the biologics within a continuous hydrogel matrix, is different from other hydrogel techniques that encapsulate cells in a homogeneous matrix. Each fibre can support a specific set of biologics and/or cell type, constituting the biostructural unit [14] , [22] ( Fig. 1b ). This primary structure can be built up into secondary structures consisting of one central fibre surrounded by other fibres, and the latter micropattern can be further repeated to form the eventual tertiary construct. In this study, prevascularised tissue constructs were formed by fibre assembly. Here an endothelial unit was surrounded by adjacent fibres encapsulating the parenchymal cells, which is in turn combined to form a construct with the aligned vasculature. The alignment of EC was achieved by presenting attachment moieties on submicron nuclear fibres within IPC fibres. These nuclear fibres aligned along the fibre axis during the drawing process [13] . RMC complexed with the nuclear fibres of the IPC fibre because of its net positive charge [23] . The presence of the aligned collagen component within the fibres helped to promote cell–matrix interaction and align cells without the use of external stimuli ( Supplementary Fig. S3 ) [23] . We applied these endothelial constructs towards engineering adipose tissue. Adipose tissue is known to be highly metabolic and susceptible to necrosis because of the lack of an oxygenated blood supply after implantation [24] , [25] , [26] . By co-patterning EC with 3T3-L1 cells in the fibre construct, we could ensure that the implanted adipose cells were in close proximity to the perfused vessels, thereby improving cell viability. Besides forming vasculature, ECs have also been shown to regulate tissue function [8] , [17] , [27] , [28] , [29] , [30] and organogenesis [31] , [32] , [33] . Thus, the functionality of 3D structures would be aided by interaction with ECs in a multicellular environment. In the case of the adipose construct, proliferation and tubulogenesis of ECs and differentiation of 3T3-L1 cells are known to be enhanced by coculture [28] , [33] . Paracrine signalling from the 3T3-L1 cells via the secretion of pro-angio-genic adipocyte-derived microvesicles further aids the formation and stabilization of microvasculature [34] . ECs have also been shown to help preserve hepatocyte function when cocultured in vitro . Patterning hepatocytes with ECs in a biomimetic sinusoid-like structure would also allow control of the geometric interaction of the hepatocytes and endothelial vessels [8] , [29] , providing a better representation of native cellular response than a random coculture [30] . The liver sinusoid-like structure thus presents a useful building block in the engineering of liver tissue. Although adipocytes and hepatocytes were the chosen parenchymal cells in the current study, a wide range of other cell types could be cultured with good viability in our tissue constructs (see Supplementary Figs S2, S3 and S4 ), and thus used in conjunction with the vascular bed. We have developed a simple and scalable technique for deriving macroscopic tissue constructs with microscopic features. This simple technique does not require specialized microfabrication equipment and can be readily adapted by most researchers. The patterned structure is obtained by simply spooling the repeat unit (secondary structure). The resolution of the construct, determined by the fibre diameter, is tunable by varying processing parameters such as the fibre draw rate, droplet size and solution concentration [13] . Moreover, sizeable constructs can be obtained from small volumes of cell suspension, with little dead volume, and within a short timespan. In this study, the generation of a single acellular construct (10 × 1 × 0.5 mm 3 ) from 50 μl of polyionic solutions typically took <15 min. Larger constructs were obtained by fusing several tertiary structures together ( Supplementary Fig. S1e ). Although chitin and alginate were used as the polyelectrolyte pair in this study, other combinations of polyelectrolytes are possible and may potentially improve tissue functionality. In conclusion, our study shows that the assembly of cell-laden polyelectrolyte hydrogel fibres is an effective prevascularisation method for creating tissue constructs. The technique enables 3D micropatterning of different cell types, in particular, the patterning of ECs to create an endothelial vessel network to support and interact with other parenchymal cells within the hydrogel. Future work will focus on applying and adapting the technology towards recapitulating the specific cell arrangements and microenvironment of various tissue types, with the eventual goal of achieving functional tissue for therapeutic applications. Fibre assembly into higher-order structures IPC fibres were drawn as previously described [13] . Five microlitre of each of WSC (1 w/v% in phosphate-buffered saline (PBS)) and alginate (1 w/v% in deionized water) solutions were dispensed on opposite sides of a pipette tip and brought into contact with each other. Fibres were then drawn by an upward motion of the tip with a linear motor at a speed of 0.3 mm s −1 . One linear motor and one rotation motor were used to assemble the fibres. Nine pairs of polyelectrolyte solution were localized on a template from which nine fibres (one central fibre with eight outer fibres) were drawn in parallel in a humidified chamber to prevent drying. Once the fibres reached a height of 5 cm, the linear motor was stopped and the base plate was rotated at 20 r.p.m. for five revolutions to allow the fibres to meet at a point. A 5-μl droplet of alginate solution (0.5 w/v%) was then applied on the fibre fusion point. Subsequently, the linear motor was reactivated to draw the fibres upwards while the droplet travelled down the nascent construct to fuse the fibres via secondary complexation. The resulting secondary structure was spooled and packed on a two-pronged collection rod, and adjacent segments of the secondary structure were fused using layer-by-layer polyelectrolyte complexation. This was performed by dipping the construct into the WSC solution (0.5 w/v%), PBS, alginate solution (0.5 w/v%) and PBS sequentially twice. The assembled tertiary structures were then removed from the collecting rod and placed in the culture medium. Encapsulation of cells and incorporation of biologics into IPC fibres For cell-laden fibres, the cells were first trypsinized and centrifuged at 500 r.p.m. for 3 min to obtain a cell pellet. The cells were taken from the pellet and mixed in the WSC solution at a cell pellet/WSC solution volume ratio of 3:7 to form a working polycation solution. This working solution was used to form IPC cell-laden fibres, and the resulting constructs were incubated in the appropriate culture medium. Biologics were incorporated by mixing in either the WSC or alginate solution. In cases where cellular alignment was required, RMC (0.25 w/v%) was added to the WSC solution ( Supplementary Methods ). Encapsulation of labelled cells HepG2 cells were subcultured in DMEM supplemented with 10 v/v% fetal bovine serum (FBS) and 1 v/v% penicillin/streptomycin (P/S). Cells were trypsinized and the cell suspension was aliquoted into two portions. Both cell suspensions were centrifuged and the supernatant was removed. Subsequently, the cells were incubated with either CellTracker Green CMFDA (10 μM) or CellTracker Orange CMTMR (10 μM) for 30 min. The supernatant was then removed and the cells were resuspended in the culture medium, followed by centrifugation to form the cell pellet. Cells stained with CellTracker Orange were encapsulated in the central fibre, whereas cells stained with CellTracker Green were encapsulated in the eight outer fibres. The tertiary construct was formed and imaged under the confocal microscope after 24 h of culture ( Fig. 1c ). Subcutaneous implantation of endothelial construct in SCID mice The animal studies were conducted in accordance to the Agency for Science, Technology and Research (A*STAR) Biological Resource Centre IACUC guidelines (Protocol No. : 090498). Human microvascular ECs (hMVECs) (third passage) and hMSC (fourth passage) (ratio 4:1) were encapsulated in the central fibre surrounded by eight cell-free fibres. The two ends of the construct were cut with a scalpel, and the constructs were then cultured in EGM2-MV medium (Lonza) for 24 h. Subsequently, we implanted the constructs (~10 × 5 × 2 mm 3 ) into mice with SCID. Mice weighing between 25 and 30 g were used without gender differentiation for the experiments. The constructs were washed thoroughly with PBS. The animals were anesthetized with ketamine (150 mg kg −1 ) and xylazine (10 mg kg −1 ) by intraperitoneal administration. The dorsum was shaved and cleansed with alternate alcohol and betadine swabs (three times). A single 0.5-cm midline incision was made using sterile surgical scalpel. Two subcutaneous pockets were created on either side of the incision. One endothelial construct and one cell-free construct (control) were implanted into each animal. The incision was closed with interrupted 4/0 sutures. For perfusion experiments, 100 μl of 5 v/v% dextran rhodamine solution (Life Technologies, USA) were injected into the tail vein of animals implanted with the constructs on Day 14 (refs 18 , 35 ). The animal was euthanized with the help of carbon dioxide inhalation after 15 min. For histological examination, the animals were killed on Days 14 and 28. For explantation, the dorsum was shaved and the previous incision was reopened. All scaffolds were retrieved with the surrounding tissue and fixed in neutral buffered formalin (10 v/v%) for processing and histological sectioning. Sections were stained with human nuclei and hVWF antibodies and counterstained with 4',6-diamidino-2-phenylindole (DAPI). Engineering prevascularised adipose tissue constructs in vivo Fibre constructs consisting of a central endothelial fibre surrounded by eight fibres with 3T3-L1 adipose precursor cells were used for implantation. After 18 days of in vitro culture in DMEM supplemented with 20% FBS, the constructs were cut with a scalpel to expose the ends of the fibre construct and washed thoroughly with PBS. The constructs were embedded in QGel, then implanted subcutaneously into SCID mice for 28 days. The explanted tissues were embedded in paraffin wax and sectioned lengthwise. Sections of cocultures were stained with H&E and oil red O. Evaluation of adipogenic differentiation in vitro Fibre constructs consisting of nine adipocyte-laden fibres were formed by suspending 3 μl of 3T3-L1 cell pellet with 7 μl of WSC, and drawing into a fibre with alginate. For coculture, the centre fibre was replaced with 3 μl of a 5:1 HUVEC:3T3-L1 cell mixture. The fibre constructs, together with a 2D tissue-culture plate control, were cultured under static culture conditions with DMEM supplemented with 10 v/v% FBS and 1 v/v% P/S for 4 days. DMEM supplemented with 20 v/v% FBS and 1 v/v% P/S was then fed to the 3T3-L1 cells for 18 days to induce adipogenesis. Differentiation of 3T3-L1 cells was indicated by the accumulation of lipid droplets. The constructs were fixed in 10% neutral buffered formalin and stained for hVWF and adiponectin to indicate the presence of ECs and differentiated adipocytes, respectively ( Supplementary Table S1 ). Engineering prevascularised hepatic tissue constructs in vivo hESCs were differentiated with a three-stage differentiation medium to obtain HPCs ( Supplementary Methods ). HUVECs (fifth passage) were encapsulated in the central fibre surrounded by eight fibres laden with HPCs. These HPC constructs were implanted at the liver injury site after partial hepatectomy in which 70% of the host liver was removed. The animals were killed on Day 14 and the explanted tissues were examined histologically. Sections of the constructs were stained with H&E and immunostained with human albumin and hCD31 antibodies ( Supplementary Table S1 ). Evaluation of primary hepatocyte constructs in vitro HUVECs (fifth passage) were encapsulated in the central fibre surrounded by eight fibres laden with primary rat hepatocytes. Hepatocyte monoculture constructs (control) were similarly created with cell-free central fibres. Hepatocyte-laden fibres were formed from polycation solution containing WSC (1 w/v%), galactosylated WSC (0.25 w/v%) and RMC (0.25 w/v%). Constructs were maintained in EndoGro-LS (Millipore) and hepatozyme-SFM (Invitrogen) (1:1 mixture) for 7 days. The medium was collected every day for albumin and urea production. Urea production was induced by incubating the constructs with culture medium supplemented with 1 mM of ammonium chloride (NH 4 Cl) for 2 h, after which the supplemented medium was removed and replaced with fresh medium. Functional maintenance of hepatocytes was assessed by measuring albumin and urea secretion over a period of 7 days ( n =3). Data for each individual construct were normalized with the Day 1 value to obtain the maintenance profiles for albumin and urea. The normalized percentages were averaged to obtain the final values. A separate experiment was conducted, whereby the hepatocyte-laden fibres did not contain galactosylated WSC. Statistical analysis All data collected were presented as mean±standard deviation (s.d.) of three samples. A Student’s t -test was used to compare the data sets. A P -value of 0.01 or less was considered statistically significant. How to cite this article: Leong, M. F. et al. Patterned prevascularised tissue constructs by assembly of polyelectrolyte hydrogel fibres. Nat. Commun. 4:2353 doi: 10.1038/ncomms3353 (2013).